Superconductivity at 5 K in alkali-metal-doped phenanthrene Organic superconductors have π -molecular orbitals, from which electrons can become delocalized, giving rise to metallic conductivity due to orbital overlap between adjacent molecules. Here we report the discovery of superconductivity at a transition temperature ( T c ) of ~5 K in alkali-metal-doped phenanthrene. A 1-GPa pressure leads to a 20% increase of T c , suggesting that alkali-metal-doped phenanthrene shows unconventional superconductivity. Raman spectra indicate that alkali-metal doping injects charge into the system to realize the superconductivity. The discovery of superconductivity in A 3 phenanthrene (where A can be either K or Rb) produces a novel broad class of superconductors consisting of fused hydrocarbon benzene rings with π-electron networks. An increase of T c with increasing number of benzene rings from three to five suggests that organic hydrocarbons with long chains of benzene rings are potential superconductors with high T c . Organic superconductors mainly belong to one of two families: the quasi-one-dimensional (TMTSF) 2 X and two-dimensional (BEDT–TTF) 2 X (refs 1 , 2 ), in which TMTSF is tetramethyltetraselenafulvalene (C 10 H 12 Se 4 ), and BEDT–TTF is bis(ethylenedithio)tetrathiafulvalene (C 10 H 8 S 8 ). The introduction of charge into C 60 solids and graphites with π-electron networks by doping to realize superconductivity has been reported [3] , [4] . Organic superconductors exhibit many interesting phenomena, including low dimensionality, strong electron–electron and electron–phonon interactions and the proximity of antiferromagnetism, insulator states and superconductivity. They consist of open-shell molecular units that are the result of a partial oxidation and reduction of the donor and acceptor molecules in the crystal-growth process. The unpaired electrons residing in the π -molecular orbital of the donor unit are responsible for the electronic properties of these charge–transfer salts. π -Molecular orbitals also have an important role in the superconductivity of C 60 solids and graphite superconductors. Key features of organic superconductors are the low dimensionality of the materials and a strong coupling of the charge carriers to the lattices. Organic superconductors provide a good system to study the interplay of strong electron–electron and electron–phonon interactions in low-dimensional system. It is striking that the close proximity of superconductivity to a magnetically ordered state occurs in organic superconductors [5] , [6] , similar to the other strongly correlated electron systems: the heavy fermion metals [7] and high-temperature superconductors including cuprates [8] and pnictides [9] , [10] . Therefore, it challenges the understanding of superconductivity. It is found that the T c increases with the expansion of the lattice in alkali-metal-doped C 60 . This behaviour is expected by the Bardeen, Cooper and Schrieffer (BCS) theory, because the expansion of lattice leads to an enhancement of the density of states on the Fermi surface. However, the body-centered-cubic fulleride Cs 3 C 60 is found to be a true Mott–Jahn–Teller insulator, and it possesses both the ingredients required by the strongly correlated theory [11] , [12] . The insulator Cs 3 C 60 can be turned into superconductor by pressure [13] . The superconductivity induced by pressure in Cs 3 C 60 is related to the antiferromagnetic Mott insulator [11] , [12] , similar to the cuprate. For the graphite superconductors with π -electron networks, C 6 Yb and C 6 Ca show superconductivity at 6.5 and 11.5 K (ref. 14 ), respectively. Such high transition temperatures are unprecedented although it is characterized by single-gap s-wave superconductivity [15] and the coupling with intercalant phonon is believed to be main force for superconductivity [16] . Therefore, it indicates that superconductivity for the superconductors with π -electron networks is not simply explained by BCS theory. Recently, a potassium-doped picene (C 22 H 14 ) with five fused benzene rings was shown to display superconductivity at a temperature as high as 18 K (ref. 17 ). Here we report the discovery of superconductivity in alkali-metal-doped phenanthrene (C 14 H 10 ). The work raises the prospect of producing a new family of superconductor based on aromatic hydrocarbons. The fact that T c increases from 5 K for A 3 phenanthrene ( A =K and Rb) with three benzene rings to 18 K for K x picene with five benzene rings suggests that organic hydrocarbons with long chains of benzene rings could be superconductors with high T c . Our results indicate that such aromatic hydrocarbons may be unconventional superconductors. 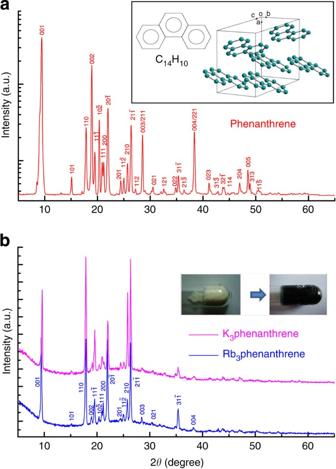Figure 1: X-ray diffraction patterns for phenanthrene andA3phenanthrene. (a) X-ray diffraction pattern for the phenanthrene purchased from Alfa Aesar. The molecular structure and crystal structure of phenanthrene are shown in the inset. (b) X-ray diffraction patterns for the superconducting samples of K3phenanthrene and Rb3phenanthrene, respectively. The inset shows the appearance for the pristine phenanthrene (white) and K3phenanthrene (black). Crystal structure of phenanthrene and A 3 phenanthrene The molecular structure and crystal structure of phenanthrene were shown in the inset of Figure 1a . Both phenanthrene and picene molecules are phenanthrene-like structure motif. The phenanthrene contains three fused benzene rings, whereas picene contains five. The ribbon-like molecular structure can be regarded as part of sheet of graphene. Figure 1a shows the X-ray diffraction pattern of phenanthrene. As shown in top panel, the phenanthrene crystallizes in P2 1 symmetry with lattice parameters: a =8.453 Å, b =6.175 Å, c =9.477 Å, β =98.28°. All peaks in X-ray diffraction pattern can be well indexed with the crystal structure mentioned above. Miller indices are marked in the pattern. The lattice constants obtained here are consistent with the results reported before [18] . The crystal that comprises layers stacked in c direction, where each layer (in a – b plane) contains phenanthrene molecules arranged in a herringbone structure, as shown in the inset of Figure 1a. Figure 1b shows the X-ray diffraction patterns of K 3 phenanthrene and Rb 3 phenanthrene with all reflections indexed with the P2 1 symmetry, and no impurity phase is observed for both K 3 phenanthrene and Rb 3 phenanthrene. Figure 1: X-ray diffraction patterns for phenanthrene and A 3 phenanthrene. ( a ) X-ray diffraction pattern for the phenanthrene purchased from Alfa Aesar. The molecular structure and crystal structure of phenanthrene are shown in the inset. ( b ) X-ray diffraction patterns for the superconducting samples of K 3 phenanthrene and Rb 3 phenanthrene, respectively. The inset shows the appearance for the pristine phenanthrene (white) and K 3 phenanthrene (black). 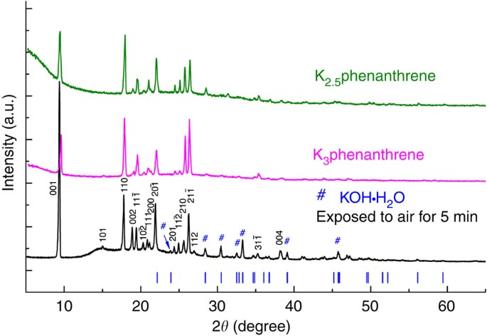Figure 2: X-ray diffraction patterns for the K3phenanthrene before and after exposing to air. Black curve was taken by putting the powder sample in Mylar film after exposing to air for 5 min to avoid more water being absorbed. The vertical short lines indicate the Bragg reflections of KOH·H2O, which appears after exposing the sample to air for 5 min. The X-ray diffraction pattern for the non-superconducting K2.5phenanthrene (green) is also shown, and all peaks can be indexed with lattice parametersa=8.449 Å,b=6.144 Å,c=9.432 Å,β=98.20°,Vcell=484.6 Å3. It seems that no big difference in structure between the superconducting and non-superconducting samples is observed. Full size image Figure 2 shows the X-ray diffraction pattern taken after exposing the superconducting K 3 phenanthrene to air for 5 min. As a comparison, the X-ray diffraction pattern for the as-grown K 3 phenanthrene is also displayed in Figure 2 . As exposed to air, the black powder products changed to white quickly. But, it should be noted that no fierce reaction, such as combustion, can be observed as exposing the as-grown K 3 phenanthrene to air, suggesting that no elementary substance of potassium remains after the reaction of potassium and phenanthrene. Figure 2 shows that the diffraction peaks of KOH·H 2 O can obviously be observed, indicating that the de-intercalation of K 3 phenantrene occurs as exposed to air, and K reacts with water to form KOH·H 2 O. The potassium de-intercalating from K 3 phenantrene in air is consistent with the fact that the K 3 phenantrene loses the superconductivity quickly for exposing to air. Such instability of K 3 phenantrene in air is quite similar to that of alkali-metal-intercalated graphite [19] , [20] , [21] and K x picene [17] . Figure 2: X-ray diffraction patterns for the K 3 phenanthrene before and after exposing to air. Black curve was taken by putting the powder sample in Mylar film after exposing to air for 5 min to avoid more water being absorbed. The vertical short lines indicate the Bragg reflections of KOH·H 2 O, which appears after exposing the sample to air for 5 min. The X-ray diffraction pattern for the non-superconducting K 2.5 phenanthrene (green) is also shown, and all peaks can be indexed with lattice parameters a =8.449 Å, b =6.144 Å, c =9.432 Å, β =98.20°, V cell =484.6 Å 3 . It seems that no big difference in structure between the superconducting and non-superconducting samples is observed. Full size image With potassium intercalated into the phenanthrene, the lattice constants of K 3 phenantrene change to a =8.430 Å, b =6.134 Å, c =9.417 Å, β =98.18 ° and the unit cell volume contracts to 482.0 Å 3 from 489.6 Å 3 . For Rb 3 phenanthrene, the lattice constants are a =8.450 Å, b =6.139 Å, c =9.442 Å, β =97.99° and the unit cell volume also contracts to 485.06 Å 3 from 489.6 Å 3 . Such contraction of lattice parameters could arise from strong interaction between the benzene ring layers induced by K or Rb doping that leads to charge transfer from dopant to the benzene rings, which is confirmed by Raman spectra. The lattice parameters of the Rb 3 phenanthrene are slightly larger than that of the K 3 phenanthrene, which arises from the fact that the ionic radius of Rb is larger than that of K. The evolution of lattice constants with K doping is quite different from the case of K x picene reported by Mitsuhashi et al . [17] , in which the remarkable feature is that the lattice constants c and b shrink, whereas the a expands with intercalating K. This is also contrary to alkali-atoms-intercalated pentacene [22] , where the lattice constant of c axis is significantly expanded because of alkali metal atoms intercalating between the molecular layers of pentacene. The intercalations in the K 3 phenanthrene and Rb 3 phenanthrene are also quite different from (BEDT–TTF) 2 I 3 (ref. 23 ) and (TMTSF) 2 PF 6 (ref. 24 ) superconductors. In superconducting (BEDT–TTF) 2 I 3 and (TMTSF) 2 PF 6 , the electron donor and acceptor layers form quasi-two-dimensional layers that is layer-by-layer stacked. 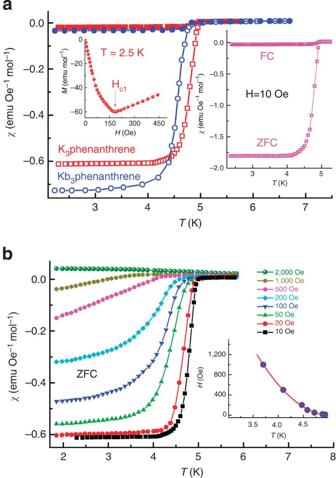Figure 3: Temperature dependence of magnetization (χ) forA3phenanthrene. (a) χ versusTplots for powder samples of K3phenanthrene withTc=4.95 K and Rb3phenanthrene withTc=4.75 K in the ZFC and FC measurements under 10 Oe, and the shield fractions are 5.3% and 6.7%, respectively. The right inset exhibits the χ versusTplot of the K3phenanthrene pellet sample by pressing powder, and a shielding fraction of 15.5% was achieved.MversusHplot for K3phenanthrene at 2.5 K was shown in the left inset. (b) χ versusTplots for the K3phenanthrene powder sample in ZFC measurements under differentH. TheHversusTcplot is shown in the inset. The onset temperature (Tconset) is defined asTc. Susceptibility of A 3 phenanthrene Figure 3a shows the magnetic susceptibility χ as a function of temperature for the powder samples of K 3 phenanthrene and Rb 3 phenanthrene in the zero-field cooling (ZFC) and field cooling (FC) measurement procedures under magnetic field H of 10Oe. The magnetic susceptibility χ versus T plot shows a sharp decrease below 4.95 K in ZFC and FC measurements for the K 3 phenanthrene, and here the temperature corresponding to the sharp decrease is defined as the superconducting transition temperature T c . One can see that the superconducting transition is very sharp and transition width is less than 0.5 K. The diamagnetic χ in the ZFC measurements can be assigned to the shielding effect, and the shielding fraction is about 5.3%. As discussed by Mitsuhashi et al . [17] , the small shielding fraction in powder sample could arise from the penetration of magnetic field into superconducting phase because of smaller size of crystallites than the London penetration depth. When the K 3 phenanthren was pressed into a pellet, the shielding fraction is increased to 15.5%. The shielding fraction of the K 3 phenanthrene is larger than that of K x picene [17] . The fact that the shielding fraction can be increased when the powder sample was pressed to form a pellet suggests that the superconductivity is a bulk behaviour. The lower critical magnetic field H C1 ~175 Oe was estimated from the M versus H plot at 2.5 K (see inset of Figure 3a ), less than H C1 ~380 Oe in K 3.3 picene with T c ~18 K at 5 K (ref. 17 ). As shown in Figure 3a , a superconducting transition at 4.75 K is observed in the susceptibility measured in ZFC and FC procedures for the powder sample Rb 3 phenanthrene with the shielding fraction of about 6.7%. It should be pointed out that T c of Rb 3 phenanthrene is about 0.20 K less than that of K 3 phenanthrene. This is consistent with the case of picene in which the T c is about 7.1 K for K doping, and shifts to 6.9 K for Rb doping. Figure 3b shows temperature dependence of χ under different magnetic fields for K 3 phenanthrene in the ZFC measurement. One can see that the diamagnetic signal disappears distinctly with increasing H , but there was an obvious drop of χ at 3.7 K even at 1,000 Oe. On the basis of data shown in Figure 3b , we obtained magnetic-field dependence of T c , and plot the upper critical field H C2 versus T in the inset of Figure 3b . Figure 3: Temperature dependence of magnetization (χ) for A 3 phenanthrene. ( a ) χ versus T plots for powder samples of K 3 phenanthrene with T c =4.95 K and Rb 3 phenanthrene with T c =4.75 K in the ZFC and FC measurements under 10 Oe, and the shield fractions are 5.3% and 6.7%, respectively. The right inset exhibits the χ versus T plot of the K 3 phenanthrene pellet sample by pressing powder, and a shielding fraction of 15.5% was achieved. M versus H plot for K 3 phenanthrene at 2.5 K was shown in the left inset. ( b ) χ versus T plots for the K 3 phenanthrene powder sample in ZFC measurements under different H . The H versus T c plot is shown in the inset. The onset temperature ( T c onset ) is defined as T c . Full size image The samples K x phenanthrene with the nominal compositions ( x =2.5, 2.8, 2.9, 3, 3.1, 3.2 and 3.5) were also synthesized in the same condition. It is found that only the sample with nominal composition K 3 phenanthrene shows superconductivity. To confirm it, we prepared five batches of samples of K x phenanthrene for the each nominal composition with x =2.5, 2.8, 2.9, 3, 3.1, 3.2 and 3.5. The parameters of superconductivity for those K x phenanthrene are displayed in Table 1 , where T c and shielding fractions were obtained from the magnetic susceptibility measurements. In the five batches of samples for each x , only the sample K x phenanthrene with the nominal composition of x =3 shows superconducting transition. Although the superconducting fraction is quite different from batch to batch among the superconducting samples, the superconducting critical temperature T c changes less than 5%. The difference of the superconducting fraction may arise from the different sizes of the crystallite. The shielding fraction from zero-field-cooled susceptibility is quite small, and the field-cooled susceptibility shows the small Meissner effect. These results could arise from the quite small size of crystallites for the powder samples, so that the penetration depth is much larger than the size of crystallites. Table 1 K x phenenthrene samples. 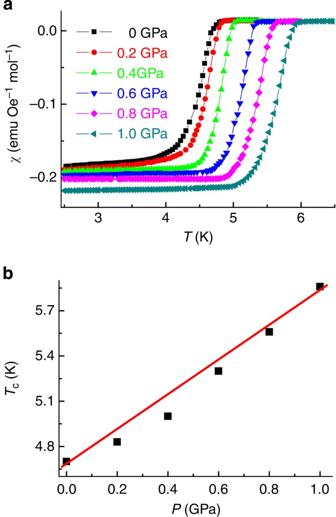Figure 4: Pressure dependence of the superconducting transitionTcfor K3phenanthrene. (a) Magnetization χ as a function of temperature for the powder sample of K3phenanthrene under the pressures ofP=0, 0.2, 0.4, 0.6, 0.8, 1.0 GPa in ZFC measurements. The sample used here was obtained by reacting phenanthrene purchased from Alfa Aesar with K. (b) Evolution ofTcwith pressure for the superconducting K3phenanthrene. Full size table Effect of pressure on T c for K 3 phenanthrene Figure 4a presents the temperature-dependent magnetization for the powder sample K x phenanthrene under the pressures ranging from ambient pressure to 1 GPa. The most notable result is that both T c and shielding fraction increase rapidly with increasing the pressure. T c is enhanced from 4.7 K at ambient pressure, to 5.9 K at 1 GPa. The pressure dependence of T c is shown in Figure 4b . The positive d (T c /T c (0))/ dP~0.26 GPa −1 at low pressure range (less than 1 GPa) in K 3 phenanthrene is similar to graphite intercalation compounds [25] . Such positive dependence would not be expected within a conventional weak coupling phonon model because T c is usually suppressed by pressure for conventional superconductivity. Figure 4: Pressure dependence of the superconducting transition T c for K 3 phenanthrene. ( a ) Magnetization χ as a function of temperature for the powder sample of K 3 phenanthrene under the pressures of P =0, 0.2, 0.4, 0.6, 0.8, 1.0 GPa in ZFC measurements. The sample used here was obtained by reacting phenanthrene purchased from Alfa Aesar with K. ( b ) Evolution of T c with pressure for the superconducting K 3 phenanthrene. 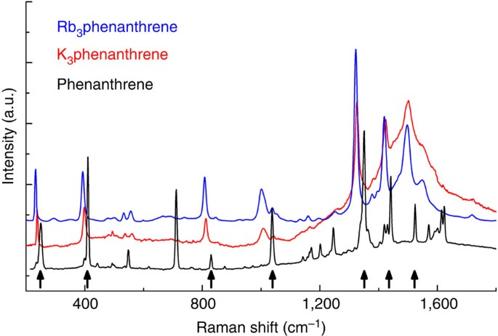Figure 5: Room temperature Raman spectra for phenanthrene andA3phenanthrene. The black arrows point to the major Raman modes with the wavelength of 1,524 cm−1, 1441 cm−1, 1,350 cm−1, 1,037 cm−1, 830 cm−1, 411 cm−1and 250 cm−1, respectively, and obvious downshift can be observed for these modes. A strong mode at 771 cm−1in pure phenanthrene becomes invisible with the potassium and rubidium intercalation. Full size image Raman spectra of phenanthrene and A 3 phenanthrene Figure 5 shows the room-temperature Raman spectra for K 3 phenanthrene and Rb 3 phenanthrene as well as pure phenanthrene. There are seven major Raman peaks, which can be conveniently compared between pure and intercalated phenanthrene: 1,524, 1,441, 1,350, 1,037, 830, 411 and 250 cm −1 , as listed in Table 2 . All of these peaks belong to the A 1 mode, and arise mainly from the C–C stretching vibration [26] , [27] . Compared with the pure phenanthrene, alkali-metal-doped phenanthrene displays obvious downshift, suggesting the phonon-mode softening effect. Such softening of the phonon modes should arise from the charge–transfer effect due to the intercalation of the alkali-metal into between phenanthrene molecules. Nominally, three electrons may transfer to a phenanthrene molecule for K 3 phenanthrene and Rb 3 phenanthrene. There are 17 and 21 cm −1 downshifts for the 1,441 cm −1 mode in K 3 phenanthrene (1424 cm −1 ) and Rb 3 phenanthrene (1,419 cm −1 ), respectively. It suggests 6 cm −1 per electron and 7 cm −1 per electron redshift with the complete transfer of charge. This is consistent with that observed in superconducting A 3 C 60 ( A =K, Rb) [28] , in which the redshift is also 6 cm −1 per electron for the mode at 1,460 cm −1 . Theoretical calculations show that the C–C stretching A 1 mode of 1,434 cm −1 (in monoanion of phenanthrene, 7 cm −1 downshift from 1441 cm −1 in the pure phenanthrene) strongly coupled to the a 2 LUMO in phenanthrene and has large electron–phonon coupling constants in the monoanion of phenanthrene [29] . The linewidth of the modes are obviously increased in K- and Rb-doped samples. Similar behaviour has been observed in potassium-doped fullerides. Such a broadening of the modes arises from the electron–phonon interaction [28] . Kato et al . have studied the electron–phonon coupling and predicted occurrence of possible superconductivity in negatively charged phenanthrene-edge-type hydrocarbon crystals based on the BCS theory with strong electron–phonon coupling [29] . They found that the strength of electron–phonon coupling and T c s have relevance to the molecular size and the molecular edge structures, and T c and electron–phonon coupling constants decrease with increasing the molecular size. Figure 5: Room temperature Raman spectra for phenanthrene and A 3 phenanthrene. The black arrows point to the major Raman modes with the wavelength of 1,524 cm −1 , 1441 cm −1 , 1,350 cm −1 , 1,037 cm −1 , 830 cm −1 , 411 cm −1 and 250 cm −1 , respectively, and obvious downshift can be observed for these modes. A strong mode at 771 cm −1 in pure phenanthrene becomes invisible with the potassium and rubidium intercalation. Full size image Table 2 The position of major Raman peaks in phenanthrene and A 3 phenanthrene. 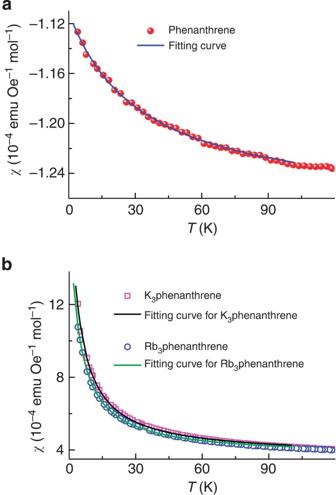Figure 6: Susceptibility of normal state for phenanthrene andA3phenanthrene. The magnetic susceptibility as a function of temperature was measured under 5 T. The fitting curves comes from the formula χ=χ0+C/(T+θ), where χ0is a constant,Cis Curie constant, andθis the paramagnetic Curie temperature. χ0is negative for pure phenanthrene while positive in the superconducting K3phenanthrene and Rb3phenanthrene. The fitting results between 4 and 80 K are listed inTable 3. Full size table Susceptibility of normal state for phenanthrene and A 3 phenanthrene We measured the magnetic susceptibility of pure phenanthrene, and superconducting K 3 phenanthrene and Rb 3 phenanthrene, as shown in Figure 6 . The magnetic susceptibilities in normal states for K 3 phenanthrene and Rb 3 phenanthrene are considerably large, and show the Curie–Weiss behaviour with the superconductivity completely suppressed under the magnetic field of 5 T. Pure phenanthrene shows diamagnetic behaviour, and the temperature-dependent negative magnetic susceptibility follows Curie–Weiss behaviour in the low-temperature regime. We fit the data of magnetic susceptibility with the formula χ=χ 0 +C/(T+θ) , and the fitting results are listed in the Table 3 . The values at 10 K for the alkali-intercalated phenanthrenes are much smaller than those reported in the superconducting K x piecene [17] . In the pure phenanthrene, only small magnetic moment of 0.06 μ B per mole is obtained from the fitting, indicating that almost no local spin is present. While in the K 3 phenanthrene and Rb 3 phenanthrene, the magnetic moment increases to 0.22 μ B per mole. It suggests that the charge transfer by the alkali intercalation into phenanthrene not only injects conduction electrons, but also induces local spins. This may hint an unconventional nature of the superconductivity in the alkali-metal-intercalated phenanthrene-edge-type hydrocarbons. Similar behaviour has been observed in K x picene. It implies that there exist local spins in these superconducting materials. It is well known that a positive pressure effect on superconductivity is widely observed in Cs 3 C 60 (ref. 11 ), high- T c cuprate compounds [30] and iron-based superconductors [31] as a consequence of the suppression of antiferromagnetism. Similar positive pressure effect on T c in aromatic hydrocarbon superconductors may also be relevant to the suppression of the localized spin interaction by pressure. Figure 6: Susceptibility of normal state for phenanthrene and A 3 phenanthrene. The magnetic susceptibility as a function of temperature was measured under 5 T. The fitting curves comes from the formula χ=χ 0 +C/(T+θ) , where χ 0 is a constant, C is Curie constant, and θ is the paramagnetic Curie temperature. χ 0 is negative for pure phenanthrene while positive in the superconducting K 3 phenanthrene and Rb 3 phenanthrene. The fitting results between 4 and 80 K are listed in Table 3 . Full size image Table 3 Fitting parameters of Curie–Weiss formula for phenanthrene and A 3 phenanthrene. Full size table We prepared a series of K x phenanthrene samples with different potassium content, and found that only the sample with nominal composition of K 3 phenanthrene shows superconductivity: all other samples with x deviation from 3 do not show superconductivity. We observed only a superconducting transition for the superconducting K 3 phenanthrene and Rb 3 phenanthrene; this is different from the case of potassium-doped picene in which there are two superconducting phases with T c =7 and 18 K, respectively. There is a large family of polycyclic aromatic compounds with an extended phenanthrene-like structural motif designated as [ n ]phenacene, where n is the number of fused benzene rings. [ n ]Phenacene molecules are related to layers of graphene in the way that ribbons are related to sheets. Therefore, discovery of superconductivity in A 3 phenanthrene ( A 3 C 14 H 10 , A =K and Rb) besides the superconductor K x picene opens a new broad family of superconductors that consists of aromatic hydrocarbons. To search for superconductors in such a family of [ n ]phenacene molecules and to study their physical properties is important to understand the mechanism of superconductivity. T c of 5 K is relatively low for A 3 phenanthrene ( A =K, Rb) with three benzene rings, compared with 7 and 18 K for K x picene with five benzene rings, suggesting that such organic hydrocarbons with long benzene rings are potential superconductors with high T c . A theoretical study by Kato et al . [29] indicates that the electron–phonon coupling constants decrease with an increase in the number of carbon atoms in phenanthrene edge-type hydrocarbons. They estimated T c for the hydrocarbon monoanions by using the approximate solution of the Eliashberg equation, and found that T c decreases with increasing the number of carbon atoms in phenanthrene edge-type hydrocarbons. However, such theoretical prediction is in contrast to experimental results, which shows that T c increases from ~5 to 7 K/18 K when increasing the number of benzene rings from 3 in phenanthrene to 5 in picene. It suggests that superconductivity in the phenanthrene edge-type hydrocarbons could be unconventional, and cannot be explained only by electron–phonon coupling. Enhancement of T c with increasing pressure and coexistence of superconductivity and local spins are also the indications of unconventional superconductivity, because the existence of local spin destroys the superconductivity in the frame of BCS theory. Further evidence for unconventional superconductivity is the decrease of T c by 0.2 K for Rb doped both phenanthrene and picene relative to K-doped samples, respectively, although the lattice constants slightly increase with change of dopant from K to Rb. This result is consistent with the pressure effect on T c . This is totally different from the case of superconducting fullerides in which T c increases with the expansion of the lattice in alkali-metal-doped C 60 (ref. 32 ), which is expected by the BCS theory, because the expansion of lattice leads to an enhancement of the density of states at the Fermi level. To confirm the proposed unconventional superconductivity, a high-quality superconducting sample, even a single crystal, may be required. This could allow the detailed determination of crystal and electronic structures and further investigation into the effects of pressure, and may reveal the mechanism of superconductivity in our organic hydrocarbon superconductors. Phenanthrene purification and sample synthesis The phenanthrene (from Alfa Aesar, 98% purity) was purified by sublimation method. The purchased phenanthrene was loaded at the bottom of a glass tube (diameter, 15 mm; length, 400 mm). The glass tube was sealed under vacuum of better than 5×10 −4 Pa. One end of the tube, where the phenanthrene was located, was put at the middle of a tubular furnace, with a thermocouple attached. The other end of the glass tube was outside of the tubular furnace. The temperature was slowly raised to 85 °C and kept for one week. The purified phenanthrene was collected at the end that was kept outside the furnace during purification. High-purity K metal (98%, Sinopharm Chemical Reagent) and phenanthrene purified by sublimation method were used as starting materials. The K metal was cut into small pieces (1 mm in diameter) and mixed with phenanthrene in the chemical stoichiometry, and then the mixture was loaded into a quartz tube (Φ=10 mm). The quartz tube was sealed under high vacuum of 1×10 −4 Pa, and then heated to 200 °C in 40 min and kept at 200 °C for 24 h. For Rb x phenanthrene samples, the mixture of Rb metal and purified phenanthrene was heated from room temperature to 240 °C in 100 min, and kept at this temperature for 7 days. At 200 °C, both phenanthrene (melting point 101 °C) and potassium (melting point 63.65 °C) are in liquid state, which can speed up the chemical reaction and insure the homogeneity of the sample. The resulting A x phenanthrene ( A =K and Rb) powder sample shows uniform dark black colour, which is totally different from the pure white colour of phenanthrene. The appearance of samples before and after annealing was shown as the inset of Figure 1b . In the Table 1 , all samples of K x phenanthrene are obtained by reacting the purified phenanthrene by sublimation method with K. The impurity phase of KH can be observed in X-ray diffraction pattern for the samples prepared by reacting the phenanthrene purchased from company with K. A x phenanthrene is quite sensitive to oxygen and moisture, and it will be decomposed in air within few minutes. All the processes except for annealing were done in glove box with the oxygen and moisture level less than 1 p.p.m. Characterization of structure and susceptibility Before the X-ray diffraction measurement, the samples were first ground into fine powder in a glove box, and then loaded into the capillaries (purchased from Hilgenberg GmbH, made of special glass no. 10. L=80 mm, OD=0.70 mm, Wall=0.01 mm); finally, the capillary was sealed to keep the sample in an inert atmosphere during X-ray diffraction measurement. The capillaries were fixed to the sample shelf of X-ray diffractometer (TTR-III theta/theta rotating anode X-ray Diffractometer) by plasticine. X-ray diffraction pattern was obtained in the 2-theta range of 5°–65° with a scanning rate of 0.5° per minute. The magnetization measurement was made by SQUID MPMS (Quantum Design). The sample was placed into Polypropylene powder holder (Quantum Design). Susceptibility under pressure The magnetization under pressure was measured by incorporating a copper–beryllium pressure cell (EasyLab) into SQUID MPMS (Quantum Design). The sample was firstly placed in a teflon cell (EasyLab) with coal oil (EasyLab) as the pressure media. Then, the teflon cell was set in the copper–beryllium pressure cell for magnetization measurement. The contribution of background magnetization against the sample at 2 K was less than 5%. Raman spectrum Raman-scattering experiments were carried out using the 780-nm laser line in DXR Raman Microscope (Thermo Scientific). The scattering light was captured with a single exposure of the CCD with a spectral resolution of 1 cm −1 . The powder samples were loaded in the sealed capillary with highly pure Ar gas during Raman measurements. It should be pointed out that the X-ray diffraction and Raman measurements were carried out on the powder samples in the same capillary. How to cite this article: Wang, X.F. et al . Superconductivity at 5 K in alkali-metal-doped phenanthrene. Nat. Commun. 2:507 doi: 10.1038/ncomms1513 (2011).